FGF signalling specifies haematopoietic stem cells through its regulation of somitic Notch signalling Haematopoietic stem cells (HSCs) derive from haemogenic endothelial cells of the primitive dorsal aorta (DA) during vertebrate embryogenesis. The molecular mechanisms governing this unique endothelial to haematopoietic transition remain unclear. Here, we demonstrate a novel requirement for fibroblast growth factor (FGF) signalling in HSC emergence. This requirement is non-cell-autonomous, and acts within the somite to bridge the Wnt and Notch signalling pathways. We previously demonstrated that Wnt16 regulates the somitic expression of two Notch ligands, deltaC ( dlc ) and deltaD ( dld ), whose combined function is required for HSC fate. How Wnt16 connects to Notch function has remained an open question. Our current studies demonstrate that FGF signalling, via FGF receptor 4 (Fgfr4), mediates a signal-transduction pathway between Wnt16 and Dlc, but not Dld, to regulate HSC specification. Our findings demonstrate that FGF signalling acts as a key molecular relay within the developmental HSC niche to instruct HSC fate. Vertebrate haematopoiesis initiates sequentially with primitive and definitive waves of blood cell production during embryogenesis [1] , [2] , [3] . Of these embryonic blood precursors, only HSCs persist into adulthood and are responsible for lifelong replenishment of the haematopoietic system. In all vertebrate animals studied, HSCs arise from haemogenic endothelium in the floor of the DA [4] , [5] . Our current understanding of HSC formation suggests that this endothelial to haematopoietic transition (EHT), which occurs during a limited window in embryonic development, gives rise to the entire pool of HSCs for the life of the organism. A major goal of regenerative medicine is to replicate the development of HSCs in vitro from human pluripotent precursors. Despite decades of effort, this goal has not been achieved. A better understanding of the molecular cues utilized by the embryo to pattern HSCs from mesodermal precursors could inform these approaches. Development of HSCs requires complex interactions between diverse molecular signalling pathways and downstream intracellular transduction networks. These pathways include Hedgehog signalling, which is required for development of endothelial progenitors and HSCs [6] , [7] , [8] , vascular endothelial growth factor (Vegf) signalling, which is critical for vasculogenesis and HSC specification [9] , [10] , [11] , bone morphogenetic protein (BMP) signalling, which specifies vascular cells from mesoderm [12] , [13] , and Notch signalling, which is essential for HSC generation from haemogenic endothelial cells [14] , [15] , [16] . The FGF signalling pathway has likewise been shown to be important in mesoderm formation [17] , [18] and vasculogenesis [19] , [20] , but only a handful of studies have addressed the role of FGF signalling in the development of the haematopoietic lineages. FGF signalling has been demonstrated to regulate formation of primitive haematopoietic cells by negatively regulating erythroid gene expression in Xenopus [21] . In the avian system, FGFs block primitive erythroid differentiation and promote endothelial development [22] . In contrast, Fgf21 knockdown in zebrafish reduced the formation of erythroid and myeloid cells [23] . In vitro studies indicated that FGFs induced myeloid proliferation in human bone marrow cultures [24] . Although the role of FGF signalling in primitive haematopoiesis has been reasonably well studied, its contribution to definitive HSC formation has never been addressed. Studies of FGF signalling and HSCs in adult mice indicate that long-term repopulating HSCs are found exclusively within an FGFR1-expressing population, and that ectopic provision of FGF1 can stimulate the in vitro expansion of HSCs [25] . However, recent in vivo studies showed that FGFR1 is not required for the homeostasis of adult HSCs but rather in the recovery of haematopoiesis following injury by enhancing HSC proliferation [26] . In this study, we utilized transgenic zebrafish in which FGF signalling can be inducibly blocked [27] . Loss of FGF signalling during early somitogenesis stages led to a loss of HSCs without disrupting development of primitive haematopoiesis or endothelium. During the temporal knockdown window, the FGF target genes pea3 and erm , as well as the receptors fgfr1 and fgfr4 , were expressed in somites but not in posterior lateral mesoderm (PLM), which includes HSC precursors. Expression of pea3 and fgfr4 was reduced following Wnt16 knockdown, which we previously showed is required for HSC emergence by its regulation of the Notch ligands dlc and dld in the developing somites [28] . Epistasis experiments demonstrated that ectopic activation of FGF signalling could rescue HSC specification in wnt16 morphants. Within the somite, FGF signalling is therefore required downstream of Wnt16 function for HSC development. Blockade of FGF signalling led to loss of dlc expression, but did not alter dld expression. Loss of HSCs following ablation of FGF signalling was restored by ectopic Notch activation. More specifically, overexpression of dlc mRNA rescued HSC emergence following loss of FGF signalling, demonstrating that FGF function is required for HSC emergence through its regulation of dlc expression. Finally, disappearance of HSCs following knockdown of Fgfr4 indicated that this receptor acts as a specific relay between Wnt16 and Dlc in the somite. Taken together, these results refine our understanding of the signalling cascades necessary within the somite to instruct HSC fate in the neighbouring PLM, and should inform studies seeking the cues necessary to pattern HSCs in vitro from pluripotent precursors. FGF signalling is required for HSC specification To examine a potential role for FGF signalling in HSC development, we used transgenic zebrafish in which FGF signalling can be conditionally abrogated by heat-shock induction of a dominant-negative Fgfr1–EGFP fusion protein ( hsp70:dn-fgfr1 ) [27] . To induce dominant-negative Fgfr1, we administered heat-shocks to transgenic animals during several different windows of development. Experimentally perturbed and wild-type (wt) embryos were examined from the outcrossed progeny of heterozygous hsp70:dn-fgfr1 fish and wt animals, resulting in 50% transgenic and 50% wt controls. As FGF signalling is critical for early vertebrate development including mesodermal patterning and somitogenesis [29] , [30] , early induction of the dn-fgfr1 transgene before 10 h post fertilization (hpf) led to gross embryonic defects ( Supplementary Fig. 1a ). However, heat induction during somitogenesis at 12 hpf (5 somites) using optimized heat-shock conditions (38 °C, 20 min) led to robust and specific loss of HSCs ( Fig. 1a–d ; Supplementary Fig. 1c ). Whole-mount in situ hybridization (WISH) with the definitive HSC markers runx1 and cmyb [31] , [32] , [33] indicated that inhibition of FGF signalling at 12 hpf led to a near complete loss of runx1 expression at 26 hpf and cmyb at 35 hpf, when compared with wt animals ( Fig. 1a–d ). Interestingly, >50% of hsp70:dn-fgfr1 transgenic embryos induced at 12 hpf showed robust loss of runx1 expression, whereas blockade of FGF signalling at 15 hpf (10 somites) or 17 hpf (15 somites) showed little alteration in runx1 expression ( Fig. 1e ). Quantitative RT-PCR (qPCR) using 26 hpf wt and hsp70:dn-fgfr1 transgenic embryos showed that runx1 expression was reduced in the absence of Fgf signalling at 12 hpf ( Supplementary Fig. 1b ). This blockade of FGF signalling at 12 hpf yielded no alteration in the number of somites during somitogenesis ( Supplementary Fig. 2h,i ), and runx1 expression in hsp70 : dn - fgfr1 transgenic embryos was similarly reduced at later developmental stages (comparing 30 hpf embryos with 26 hpf embryos; Supplementary Fig. 1d ), suggesting that loss of HSCs following FGF blockade was not caused by aberrant developmental rate. We further quantified the number of cmyb + HSCs in the DA (yellow arrowheads in Fig. 1c,d ) and observed that FGF signalling inhibition at 12 hpf, but not at later time points, perturbed HSC formation, consistent with our runx1 analyses ( Fig. 1f ). Further quantification of emerging HSCs using triple transgenic cmyb:EGFP; kdrl:RFP; hsp70:dn-fgfr1 embryos demonstrated that cmyb + kdrl + double-positive HSCs were significantly reduced after heat induction at 12 hpf compared with wt ( Fig. 1g–i ). In addition, at 4 and 5 days post fertilization (dpf), expression of cmyb and rag1 , markers of developing T lymphocytes in the thymus, was largely lost following the ablation of FGF signalling at 12 hpf ( Fig. 1j–m ). Since thymocyte production requires upstream HSCs, these results indicate that FGF signalling is required for HSC development. 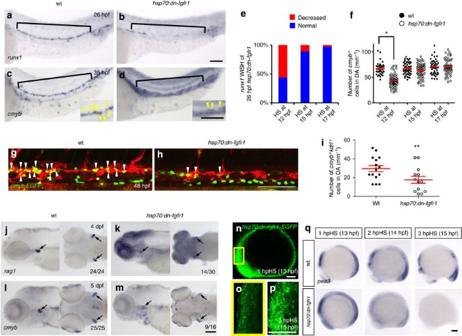Figure 1: FGF signalling is required for HSC specification during mid-somitogenesis stages. (a–d)hsp70:dn-fgfr1transgenic embryos, heat induced at 12 hpf (38 °C, 20 min) visualized by WISH for HSC markersrunx1(black brackets) (a,b) andcmyb(black brackets and yellow arrowheads in high magnification images) (c,d) in aortic haemogenic endothelium compared with wt embryos. (e)runx1phenotype percentages inhsp70:dn-fgfr1animals following heat-shock at the indicated stages (12 hpf,n=82; 15 hpf,n=26;17 hpf,n=38). (f) Quantification of 35 hpfcmyb+cells (yellow arrowheads inc,d) in the DA of wt andhsp70:dn-fgfr1induced at 12 hpf (wt,n=42;hsp70:dn-fgfr1,n=61; *P-value<0.00001, significantly different from wt, Student’st-test), 15 hpf (wt,n=52;hsp70:dn-fgfr1,n=56), and 17 hpf (wt,n=48;hsp70:dn-fgfr1,n=54). Red lines indicate mean±s.e.m. (g,h) Confocal microscopy images of 48 hpf double-positive HSCs (white arrowheads) incmyb:EGFP; kdrl;RFP; hsp70:dn-fgfr1animals following heat-shock at 12 hpf. (i) Quantification of 48 hpfcmyb+kdrl+double-positive HSCs in the DA of wt andhsp70:dn-fgfr1animals induced at 12 hpf (wt,n=15;hsp70:dn-fgfr1,n=13; **P-value<0.005, significantly different from wt, Student’st-test). (j–m) Lateral and ventral view of WISH images usinghsp70:dn-fgfr1transgenic embryos heat-induced at 12 hpf forrag1at 4 dpf (j,k) andcmybat 5 dpf (l,m) in thymus (black arrows) compared with wt embryos. (n–p) Confocal microscopy images ofhsp70:dn-fgfr1embryos heat-shocked at 12 hpf. Expression of dominant-negative Fgfr1-EGFP at 13 hpf (n,o) and 15 hpf (p). (o) The magnified region boxed in yellow shown in (n). (q) WISH for the FGF targetpea3in wt (top row) andhsp70:dn-fgfr1embryos (bottom row) at 13, 14, and 15 hpf after heat-shock at 12 hpf. Scale bar=100 μm. Figure 1: FGF signalling is required for HSC specification during mid-somitogenesis stages. ( a – d ) hsp70:dn-fgfr1 transgenic embryos, heat induced at 12 hpf (38 °C, 20 min) visualized by WISH for HSC markers runx1 (black brackets) ( a , b ) and cmyb (black brackets and yellow arrowheads in high magnification images) ( c , d ) in aortic haemogenic endothelium compared with wt embryos. ( e ) runx1 phenotype percentages in hsp70:dn-fgfr1 animals following heat-shock at the indicated stages (12 hpf, n =82; 15 hpf, n =26;17 hpf, n =38). ( f ) Quantification of 35 hpf cmyb + cells (yellow arrowheads in c , d ) in the DA of wt and hsp70:dn-fgfr1 induced at 12 hpf (wt, n =42; hsp70:dn-fgfr1 , n =61; * P -value<0.00001, significantly different from wt, Student’s t -test), 15 hpf (wt, n =52; hsp70:dn-fgfr1 , n =56), and 17 hpf (wt, n =48; hsp70:dn-fgfr1 , n =54). Red lines indicate mean±s.e.m. ( g , h ) Confocal microscopy images of 48 hpf double-positive HSCs (white arrowheads) in cmyb:EGFP; kdrl;RFP; hsp70:dn-fgfr1 animals following heat-shock at 12 hpf. ( i ) Quantification of 48 hpf cmyb + kdrl + double-positive HSCs in the DA of wt and hsp70:dn-fgfr1 animals induced at 12 hpf (wt, n =15; hsp70:dn-fgfr1 , n =13; ** P -value<0.005, significantly different from wt, Student’s t -test). ( j – m ) Lateral and ventral view of WISH images using hsp70:dn-fgfr1 transgenic embryos heat-induced at 12 hpf for rag1 at 4 dpf ( j , k ) and cmyb at 5 dpf ( l , m ) in thymus (black arrows) compared with wt embryos. ( n – p ) Confocal microscopy images of hsp70:dn-fgfr1 embryos heat-shocked at 12 hpf. Expression of dominant-negative Fgfr1-EGFP at 13 hpf ( n , o ) and 15 hpf ( p ). ( o ) The magnified region boxed in yellow shown in ( n ). ( q ) WISH for the FGF target pea3 in wt (top row) and hsp70:dn-fgfr1 embryos (bottom row) at 13, 14, and 15 hpf after heat-shock at 12 hpf. Scale bar=100 μm. Full size image To more precisely determine the critical time window that FGF signalling affects HSC formation, we investigated the expression of dominant-negative Fgfr1-EGFP fusion proteins by confocal microscopy. Membrane-localized EGFP was observed within an hour of heat-shock ( Fig. 1n,o ) and robustly expressed by 3 h ( Fig. 1p ). In parallel, we also examined expression of a known target of FGF signalling, pea3 (refs 34 , 35 ) ( Fig. 1q ). Concomitant with the expression of dominant negative Fgfr1–EGFP fusion protein, pea3 expression was severely reduced at 2 h post heat-shock (hpHS), and absent by 3 hpHS. Taken together, these data indicate that the temporal developmental window where FGF signalling is required to specify HSCs is during mid-somitogenesis between 14 and 17 hpf. To determine whether failure of HSC specification in induced hsp70:dn-fgfr1 animals was due to incorrect specification of other mesodermal tissues, we examined expression of the PLM markers scl , fli1 and lmo2 at 15 hpf ( Fig. 2a,b ; Supplementary Fig. 2a,b ), the ventral mesoderm marker cdx4 ( Fig. 2c,d ), the notochord marker shh and its targets ptc1 and ptc2 ( Fig. 2e,f ; Supplementary Fig. 2c,d ), the somitic markers desma and vegfa ( Fig. 2g,h ; Supplementary Fig. 2g ), the primitive erythrocyte marker, gata1 ( Fig. 2k,l ), and a pan-leukocyte marker, l-plastin ( Fig. 2m,n ). We observed no gross alterations in any of these tissues or cells. Similarly, convergence of pre-haematopoietic mesoderm was not significantly affected ( Fig. 2i,j ; Supplementary Fig. 2j ). Importantly, expression of the pan-vascular markers kdrl, fli1 and cdh5 was normal at 26 hpf ( Fig. 2o–r : Supplementary Fig. 2f,k ), as was efnb2a , a marker of aortic fate commitment ( Fig. 2s,t ; Supplementary Fig. 2k ), indicating that the observed HSC defects are not likely a result of improper aortic specification. 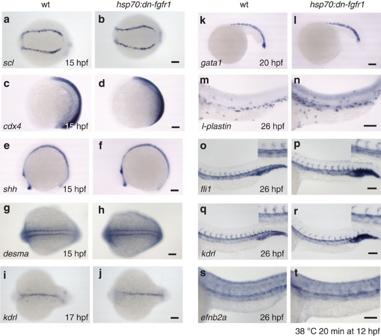Figure 2: The effect of FGF signalling on HSC formation is specific. WISH of wt and inducedhsp70:dn-fgfr1at 12 hpf with the PLM markerscl(a,b) at 15 hpf, the ventral mesoderm markercdx4at 15 hpf (c,d), the floorpalate and notochord markershhat 15 hpf (e,f) and the somite markerdesmaat 15 hpf (g,h), the endothelial markerkdrlat 17 hpf (i,j), the primitive erythroid markergata1at 20 hpf (k,l), the primitive leukocyte markerl-plastinat 26 hpf (m,n), the endothelial markersfli1andkdrlat 26 hpf (o–r; expression in the aorta and vein with higher magnification included), and the arterial markerefnb2aat 26 hpf (s,t). Scale bar=100 μm. Figure 2: The effect of FGF signalling on HSC formation is specific. WISH of wt and induced hsp70:dn-fgfr1 at 12 hpf with the PLM marker scl ( a , b ) at 15 hpf, the ventral mesoderm marker cdx4 at 15 hpf ( c , d ), the floorpalate and notochord marker shh at 15 hpf ( e , f ) and the somite marker desma at 15 hpf ( g , h ), the endothelial marker kdrl at 17 hpf ( i , j ), the primitive erythroid marker gata1 at 20 hpf ( k , l ), the primitive leukocyte marker l-plastin at 26 hpf ( m , n ), the endothelial markers fli1 and kdrl at 26 hpf ( o – r ; expression in the aorta and vein with higher magnification included), and the arterial marker efnb2a at 26 hpf ( s , t ). Scale bar=100 μm. Full size image FGF signalling is active in the somites but not in the PLM On refining the temporal window in which FGF signalling was required for HSC specification, we investigated what tissues were receiving FGF signals in this time frame to determine whether or not HSC specification might require FGF cell autonomously. First, we examined expression of the FGF targets pea3 and erm at 15 hpf and observed that their expression localized mainly to somites ( Supplementary Fig. 3 ). To more precisely determine the expression pattern of FGF target genes, we utilized two-colour enzymatic or fluorescence WISH (FISH) using pea3 and erm along with markers of PLM, which contains the precursors of HSCs [5] , [36] , [37] , [38] ( Fig. 3a,d–f ). Expression of pea3 and erm was restricted primarily to the somites and pre-somitic mesoderm, and did not overlap with fli1 + or lmo2 + PLM at 15 hpf, indicating that FGF signalling required for HSC specification is active in somites but not in the pre-endothelial mesoderm. 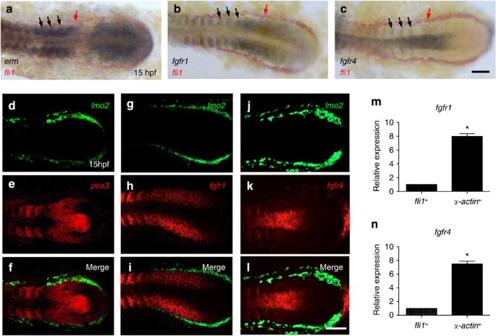Figure 3: FGF signalling is active in somitic tissues but not in the pre- endothelial PLM during mid-somitogenesis. (a–c) Images of double enzymatic WISH using probes for the FGF target geneerm(a),fgfr1(b), andfgfr4(c) expressed in somites (black arrows) and the PLM markerfli1(red arrows) at 15 hpf. (d–l) Confocal images of two-colour FISH with the PLM markerlmo2(green ind,g,j), fgfr1, fgfr4and the FGF target genepea3(red ine,h,k) and merged images (f,i,l). (m,n) qPCR expression of pre-endothelial PLMfli1:EGFP+cells and somite-specificα-actin:GFP+cells at 17 hpf. Expression data were normalized toef1αlevels (α-actin+fraction,n=3; *Pvalue<0.005, significantly different fromfli1+, Student’st-test). Scale bar=100 μm. Figure 3: FGF signalling is active in somitic tissues but not in the pre- endothelial PLM during mid-somitogenesis. ( a – c ) Images of double enzymatic WISH using probes for the FGF target gene erm ( a ), fgfr1 ( b ), and fgfr4 ( c ) expressed in somites (black arrows) and the PLM marker fli1 (red arrows) at 15 hpf. ( d – l ) Confocal images of two-colour FISH with the PLM marker lmo2 (green in d , g , j ) , fgfr1, fgfr4 and the FGF target gene pea3 (red in e , h , k ) and merged images ( f , i , l ). ( m , n ) qPCR expression of pre-endothelial PLM fli1:EGFP + cells and somite-specific α-actin:GFP + cells at 17 hpf. Expression data were normalized to ef1α levels ( α-actin + fraction, n =3; * P value<0.005, significantly different from fli1 + , Student’s t -test). Scale bar=100 μm. Full size image As FGF signalling is transduced by dimerized ligand-bound FGFRs [39] , identifying the spatial distribution of individual receptors provides excellent resolution as to which cells are experiencing FGF signalling in addition to the expression of FGF targets. We examined the expression of all four FGFRs at 15 hpf utilizing WISH and observed no receptor expression in the PLM ( Supplementary Fig. 3 ). In particular, fgfr2 and fgfr3 were not expressed in the embryo posterior, whereas fgfr1 and fgfr4 were expressed in the posterior somites, similar to the FGF targets pea3 and erm . Two-colour WISH using probes against fgfr1 or fgfr4 and the PLM marker fli1 or lmo2 also demonstrated that neither receptor was expressed in the fli1 + or lmo2 + PLM tissue ( Fig. 3b,c,g–l ). In addition to whole-animal imaging approaches, we purified PLM precursors ( fli1 + ) and somitic cells ( α-actin + ) from 17 hpf fli1:EGFP or α-actin:GFP transgenic embryos by fluorescence-activated cell sorting (FACS) to query expression of fgfr1 and fgfr4 by qPCR. Consistent with our WISH and FISH results, expression of fgfr1 and fgfr4 segregated to the somite fractions ( Fig. 3m,n ). Taken together, these data suggest that FGF signalling does not act directly on HSC precursors and the requirement for FGF signalling is non-cell autonomous. Wnt16 acts upstream of FGF signalling in HSC specification Recent studies from our laboratory showed that Wnt16 regulates the somitic expression of the Notch ligands dlc and dld whose combined activity is required to specify HSCs during somitogenesis [28] ( Supplementary Fig. 5a ). On the basis of spatiotemporal similarities between Wnt16 and FGF activity, we hypothesized the existence of a Wnt16/FGF regulatory network in the somite between 14 and 17 hpf. To test this hypothesis, we first examined the expression of wnt16 and the FGF target pea3 . As we have seen previously [28] , wnt16 transcript was localized to a relatively anterior-dorsal-lateral compartment of each of the more rostral somites. pea3 was expressed in the anterior-lateral compartment of more posterior somites, as well as the presomitic mesoderm (PSM) ( Fig. 4a–e ). As the perdurance and signalling range of Wnt16 protein is unknown, it is difficult to determine whether Wnt16 has a role in somitic maintenance of pea3 expression that initiates in the PSM. To further analyse potential epistasis between Wnt16 and FGFs, we knocked down wnt16 with an antisense-morpholino (wnt16-MO) and assessed pea3 expression ( Fig. 4f,g ; Supplementary Fig. 4 ). Expression of pea3 was robustly downregulated in the formed somites at 17 hpf in the absence of Wnt16, although PSM expression was unaffected. These results indicate that Wnt16 regulates somitic FGF signalling within our noted HSC specification time window. Furthermore, expression of fgfr4 was reduced in wnt16 morphants, while fgfr1 was unchanged relative to control embryos ( Fig. 4h,i ; Supplementary Figs 4 and 5a ). To confirm that Wnt16 acts upstream of FGF signalling to specify HSCs, we utilized a heat-inducible gain-of-function animal carrying a constitutively-active Fgfr1 transgene ( hsp70:ca-fgfr1 ) [40] . Ectopic activation of FGF signalling at 12 hpf recovered normal runx1 expression in the DA at 26 hpf, as well as pea3 expression at 17 hpf in wnt16 morphants ( Fig. 4j–n ; Supplementary Fig. 5b ). Uninjected but heat-shocked hsp70:ca-fgfr1 animals showed no ectopic increase in runx1 expression ( Fig. 4k ). Similar to the early somitic requirements for Wnt16 and FGF in HSC specification, Vegf signalling is known to function in the development of the vasculature and definitive HSCs during somitogenesis [9] , [10] , [11] . To determine whether Vegf signalling also regulates the activity of FGF signalling, we treated embryos with the Vegf inhibitor ZM306416 during somitogenesis. In contrast to the observed epistasis between Wnt16 and FGF signalling in the somites, pharmacological inhibition of Vegf signalling produced no alteration in expression of either pea3 or fgfr4 in the somites compared with DMSO-treated controls ( Supplementary Fig. 5c, d ). Taken together, these results suggest that Wnt16 regulates the FGF signalling pathway during somitogenesis to specify HSCs. 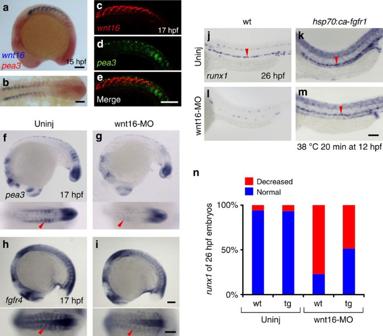Figure 4: Wnt16 controls FGF signalling activity. (a,b) Expression ofwnt16(blue) andpea3(red) at 15 hpf by two-colour enzymatic whole-mount and flat-mountin situhybridization. (c–e) Confocal images of FISH forwnt16(red inc),pea3(green ind), or merge (e) at 17 hpf. (f–i) Lateral and dorsal views of expression ofpea3(f,g) andfgfr4(h,i) inwnt16morphants at 17 hpf compared with uninjected controls as indicated at top. (j–m) WISH forrunx1expression at 26 hpf following ectopic activation of FGF signalling usinghsp70:ca-fgfr1induced at 12 hpf (38 °C 20 min) inwnt16morphants. (n)runx1phenotype percentages in wnt16-MO injectedhsp70:ca-fgfr1transgenic embryos (tg) heat-shocked at 12 hpf, compared with wnt16-MO injected wt embryos (uninjected wt,n=34; uninjected tg,n=44; wnt16-MO injected wt,n=48; wnt16-MO injected tg,n=37). Red arrowheads indicate WISH signals ofpea3andfgfr4in the somites (f–i) andrunx1in the DA (j–m). Scale bar=100 μm. Figure 4: Wnt16 controls FGF signalling activity. ( a , b ) Expression of wnt16 (blue) and pea3 (red) at 15 hpf by two-colour enzymatic whole-mount and flat-mount in situ hybridization. ( c – e ) Confocal images of FISH for wnt16 (red in c ), pea3 (green in d ), or merge ( e ) at 17 hpf. ( f – i ) Lateral and dorsal views of expression of pea3 ( f , g ) and fgfr4 ( h , i ) in wnt16 morphants at 17 hpf compared with uninjected controls as indicated at top. ( j – m ) WISH for runx1 expression at 26 hpf following ectopic activation of FGF signalling using hsp70:ca-fgfr1 induced at 12 hpf (38 °C 20 min) in wnt16 morphants. ( n ) runx1 phenotype percentages in wnt16-MO injected hsp70:ca-fgfr1 transgenic embryos (tg) heat-shocked at 12 hpf, compared with wnt16-MO injected wt embryos (uninjected wt, n =34; uninjected tg, n =44; wnt16-MO injected wt, n =48; wnt16-MO injected tg, n =37). Red arrowheads indicate WISH signals of pea3 and fgfr4 in the somites ( f – i ) and runx1 in the DA ( j – m ). Scale bar=100 μm. Full size image Somitic expression of dlc but not dld requires FGF signalling Previous studies suggest that FGF signalling can control Notch ligand expression in the somites through regulation of the transcription factor FoxD5 (ref. 41 ). Our previous work showed that Wnt16 is required for dlc and dld expression [28] , but how this regulation is mediated is unknown. Our results above indicate that Wnt16 acts upstream of FGF signalling in HSC specification, suggesting the possibility that FGF signalling might be required for dlc and dld expression. We therefore tested whether FGF signalling might regulate somitic expression of dlc and/or dld . To investigate this question, we blocked FGF signalling with a 12 hpf induction of hsp70:dn-fgfr1 transgenic animals followed by WISH for dlc and dld at 15 hpf. Loss of FGF signalling led to a loss of somitic dlc expression at 15 hpf ( Fig. 5a,b ). Likewise, the sclerotome marker foxc1b , which requires somitic Dlc [28] , was reduced in the absence of FGF signalling ( Supplementary Fig. 6a ). This effect was specific to the somites, as expression of other Notch ligands and receptors, including dlc in endothelium at 26 hpf, was not altered ( Supplementary Fig. 6b ). In addition, pharmacological inhibition using the FGFR antagonist SU5402 led to a robust reduction of dlc expression when compared with DMSO-treated controls, whereas ectopic activation of FGF signalling enhanced dlc expression in the somites ( Fig. 5c,d ; Supplementary Fig. 6c ). In contrast to the effects of dlc , somitic expression of dld was not altered following loss of FGF signalling ( Fig. 5e–h ), indicating that FGF is dispensable for dld expression but required specifically for somitic dlc expression. 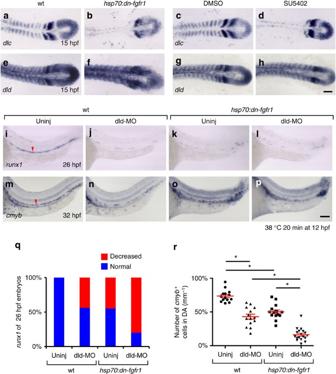Figure 5: Somiticdlcexpression, but notdld, is regulated by FGF signalling. (a–h) Expression of Notch ligandsdlcanddldin 15 hpfhsp70:dn-fgfr1animals heat-shocked at 12 hpf compared with wt controls (a,b,e,f) and wt embryos incubated with the FGFR-antagonist SU5402 (12–15 hpf) compared with DMSO-treated controls (c,d,g,h). (i–p) Expression of HSC markersrunx1at 26 hpf (i–l) andcmybat 32 hpf (m–p) in uninjected wt (i,m), dld-MO injected wt (j,n), uninjectedhsp70:dn-fgfr1(k,o) and dld-MO injectedhsp70:dn-fgfr1(l,p) embryos heat-shocked at 12 hpf. Red arrowheads indicaterunx1orcmybWISH signals in uninjected controls (i,m). (q,r) Percentage of embryos displaying arunx1phenotype at 26 hpf (q; uninjected wt,n=54; dld-MO injected wt,n=41; uninjectedhsp70:dn-fgfr1,n=58; dld-MO injectedhsp70:dn-fgfr1,n=45) and quantification ofcmyb+cells in DA (r; uninjected wt,n=14; dld-MO injected wt,n=14; uninjectedhsp70:dn-fgfr1,n=15; dld-MO injectedhsp70:dn-fgfr1,n=18; mean±s.e.m.; *P<0.00001, Student’st-test) after blockingdldexpression and FGF signalling. Scale bar=100 μm. Figure 5: Somitic dlc expression, but not dld , is regulated by FGF signalling. ( a – h ) Expression of Notch ligands dlc and dld in 15 hpf hsp70:dn-fgfr1 animals heat-shocked at 12 hpf compared with wt controls ( a , b , e , f ) and wt embryos incubated with the FGFR-antagonist SU5402 (12–15 hpf) compared with DMSO-treated controls ( c , d , g , h ). ( i – p ) Expression of HSC markers runx1 at 26 hpf ( i – l ) and cmyb at 32 hpf ( m – p ) in uninjected wt ( i , m ), dld-MO injected wt ( j , n ), uninjected hsp70:dn-fgfr1 ( k , o ) and dld-MO injected hsp70:dn-fgfr1 ( l , p ) embryos heat-shocked at 12 hpf. Red arrowheads indicate runx1 or cmyb WISH signals in uninjected controls ( i , m ). ( q , r ) Percentage of embryos displaying a runx1 phenotype at 26 hpf ( q ; uninjected wt, n =54; dld-MO injected wt, n =41; uninjected hsp70:dn-fgfr1 , n =58; dld-MO injected hsp70:dn-fgfr1 , n =45) and quantification of cmyb + cells in DA ( r ; uninjected wt, n =14; dld-MO injected wt, n =14; uninjected hsp70:dn-fgfr1 , n =15; dld-MO injected hsp70:dn-fgfr1 , n =18; mean±s.e.m. ; * P <0.00001, Student’s t -test) after blocking dld expression and FGF signalling. Scale bar=100 μm. Full size image Combined expression of dlc and dld is required for HSC specification downstream of Wnt16, whereas single knockdown of either ligand incompletely blocked HSC formation [28] . We therefore reasoned that the incomplete loss of HSCs following loss of FGF signalling ( Fig. 1e ) may be due to residual somitic Notch signalling mediated by dld. We therefore tested whether or not combined loss of Dld and FGF function would lead to a more complete loss of HSCs. We analysed the expression of runx1 (26 hpf) and cmyb (32 hpf) in dld-MO injected hsp70:dn-fgfr1 and wt control embryos heat-shocked at 12 hpf ( Fig. 5i–p ). Whereas injection of individual dld-MO into wt embryos led to a loss of runx1 and cmyb expression at levels comparable to heat-induced hsp70:dn-fgfr1 alone, combinatorial ablation of FGF signalling and Dld function led to significantly lower numbers of HSCs ( Fig. 5q,r ). Finally, to confirm that FGF signalling acts upstream of dlc to specify HSCs, we performed rescue experiments in which hsp70:dn-fgfr1 animals were injected with dlc mRNA at the 1-2-cell stage of development followed by heat-shock at 12 hpf. As assessed by runx1 and cmyb expression, HSC numbers were significantly rescued following injection of dlc in the absence of FGF signalling ( Fig. 6a–f ; Supplementary Fig. 7a ). To examine this in another way, we performed rescue experiments with transgenic animals whereby Notch signalling can be experimentally activated by heat induction ( hsp70:gal4; UAS:NICD-myc ) [14] , [42] . To obtain triple transgenic animals, hsp70:dn-fgfr1 animals were crossed with hsp70:gal4; UAS:NICD-myc fish. Both dn-Fgfr1 and NICD-myc, transgenes were induced by heat-shock at 12 hpf, and NICD + transgenic fish were identified by myc-antibody staining after runx1 WISH was performed ( Supplementary Fig. 7c ). NICD overexpression in hsp70:dn-fgfr1 embryos led to a mild recovery of runx1 expression ( Supplementary Fig. 7b,d ). As heat-shock at later time points (15 hpf) showed no loss of HSCs in hsp70 : dn - fgfr1 embryos ( Fig. 1e,f ), we performed a second heat-shock in triple transgenic embryos to maximize the effects of NICD on HSC specification. A first heat-shock was administered at 12 hpf to ablate FGF signalling by 15 hpf. Next, a second heat-induction was performed at 14 hpf, as this time point was previously utilized to optimally rescue HSC specification in wnt16 morphants via NICD induction [28] . WISH for runx1 at 26 hpf demonstrated that activation of Notch signalling almost fully recovered runx1 + HSCs following ablation of FGF signalling ( Fig. 6g–m ). Taken together, these results demonstrate that FGF signalling is required for dlc but not dld expression in somites to regulate HSC specification during somitogenesis. 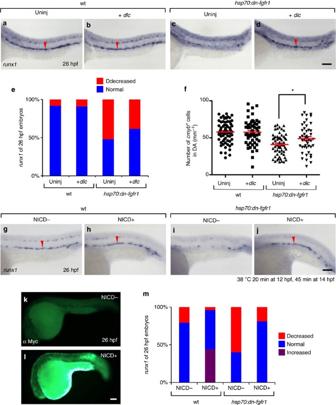Figure 6: FGF regulation of HSC specification requires the Notch ligand Dlc. (a–d) Expression ofrunx1in wt andhsp70:dn-fgfr1embryos injected with 100 pg ofdlcmRNA and uninjected controls. Embryos were heat induced at 12 hpf. (e,f) Quantitation of defective embryos showing decreased expression ofrunx1at 26 hpf (e; uninjected wt,n=61;dlc+wt,n=44; uninjectedhsp70:dn-fgfr1,n=46;dlc+hsp70:dn-fgfr1,n=52) andcmyb+cells at 32 hpf (f; uninjected wt,n=68;dlc+wt,n=56; uninjectedhsp70:dn-fgfr1,n=58;dlc+hsp70:dn-fgfr1,n=46) usinghsp70:dn-fgfr1injected withdlcmRNA and followed by heat-shock at 12 hpf (mean±s.e.m.; *P<0.05, Student’st-test). (g–j)runx1expression at 26 hpf inhsp70:gal4; UAS:NICD-myc; hsp70:dn-fgfr1heat-shocked at both 12 and 14 hpf. (k,l) NICD+ embryos were identified by immunostaining for the myc epitope tag, following WISH. (m) Percentage of embryos with arunx1phenotype at 26 hpf in wt or FGF-blocked, with or without enforced NICD expression (NICD- wt,n=48; NICD+ wt,n=25; NICD-hsp70:dn-fgfr1,n=20; NICD+hsp70:dn-fgfr1,n=21). Red arrowheads indicaterunx1expression in the DA. Scale bar=100 μm. Figure 6: FGF regulation of HSC specification requires the Notch ligand Dlc. ( a – d ) Expression of runx1 in wt and hsp70:dn-fgfr1 embryos injected with 100 pg of dlc mRNA and uninjected controls. Embryos were heat induced at 12 hpf. ( e , f ) Quantitation of defective embryos showing decreased expression of runx1 at 26 hpf ( e ; uninjected wt, n =61; dlc +wt, n =44; uninjected hsp70:dn-fgfr1 , n =46; dlc + hsp70:dn-fgfr1 , n =52) and cmyb + cells at 32 hpf ( f ; uninjected wt, n =68; dlc +wt, n =56; uninjected hsp70:dn-fgfr1 , n =58; dlc + hsp70:dn-fgfr1 , n =46) using hsp70:dn-fgfr1 injected with dlc mRNA and followed by heat-shock at 12 hpf (mean±s.e.m. ; * P <0.05, Student’s t -test). ( g – j ) runx1 expression at 26 hpf in hsp70:gal4; UAS:NICD-myc; hsp70:dn-fgfr1 heat-shocked at both 12 and 14 hpf. ( k , l ) NICD+ embryos were identified by immunostaining for the myc epitope tag, following WISH. ( m ) Percentage of embryos with a runx1 phenotype at 26 hpf in wt or FGF-blocked, with or without enforced NICD expression (NICD- wt, n =48; NICD+ wt, n =25; NICD- hsp70:dn-fgfr1 , n =20; NICD+ hsp70:dn-fgfr1 , n =21). Red arrowheads indicate runx1 expression in the DA. Scale bar=100 μm. Full size image Fgfr4 acts to relay Wnt16 signals to Dlc to specify HSCs During early to mid-somitogenesis, knockdown of Wnt16 led to diminished expression of fgfr4 but no alteration of fgfr1 in somites ( Fig. 4h,i ; Supplementary Fig. 5a ). Moreover, two-colour FISH demonstrated that dlc was expressed in fgfr4 + but not in fgfr1 + somitic tissues ( Fig. 7a–f ). On the basis of these results, we hypothesized that Fgfr4 may mediate the Wnt16/Dlc signalling cascade to regulate HSC specification. To test this hypothesis, we knocked down the function of fgfr4 using both splicing-blocking (fgfr4-MO1) and translation-blocking (fgfr4-MO2) receptor-specific MOs. We observed that dlc expression in somites at 15 hpf as well as foxc1b expression in the sclerotome was reduced in both fgfr4 morphants when compared with uninjected and control MO-injected embryos ( Fig. 7g–i ; Supplementary Figs 4 and 8b ). By contrast, knockdown of fgfr1 led to no alteration in dlc expression ( Supplementary Fig. 8a ). Finally, to determine whether regulation of dlc via Fgfr4 is upstream of HSC generation, we analysed HSC marker expression in fgfr4 morphants. Loss of Fgfr4 function led to a marked decrease in the number of runx1 + and cmyb + cells along the DA ( Fig. 7j–o ; Supplementary Fig. 8b,c ). Although fgfr4 morphant animals showed slight patterning defects potentially caused by the ablation of fgfr4 at earlier developmental stages [43] , both endothelium and DA appeared normal in the morphants ( Fig. 7p–u ; Supplementary Fig. 8b ). In addition, knock down of fgfr4 using fgfr4-MO2 led to no alterations in shh and vegf expression, whereas expression of the sclerotomal marker foxc1b was severely reduced ( Supplementary Fig. 8d ), consistent with our findings in hsp70 : dn - fgfr1 transgenic animals ( Fig. 2e,f ; Supplementary Fig. 2g and 6a ). Further analysis of HSC emergence using cmyb:EGFP; kdrl:RFP transgenic animals [5] showed a marked reduction in the number of cmyb + kdrl + double-positive HSCs in fgfr4 morphants compared with controls ( Fig. 7v–y ). Taken together, these results indicate that Fgfr4 plays a pivotal role in mediating the Wnt16/Dlc signalling cascade required for instruction of HSC fate. 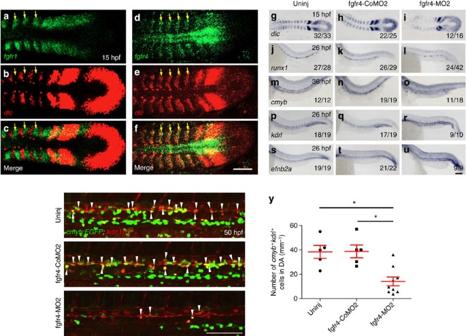Figure 7: Fgfr4 is required for somiticdlcexpression and HSC specification. (a–f) Single-plane confocal images of two-colour FISH forfgfr1(a),dlc(b) and merged comparison (c), andfgfr4(d),dlc(e) and their merged comparison (f) at 15 hpf. Yellow arrows indicate expressions offgfr1(a) orfgfr4(d) in the somites. (g–u) Expression of somiticdlcat 15 hpf. (g–i),runx1at 26 hpf (j–l),cmybat 36 hpf (m–o), the endothelium markerkdrl(p–r) and the aortic markerefnb2a(s–u) at 26 hpf in fgfr4-MO2 injected embryos, compared with uninjected and mismatched control MO (fgfr4-CoMO2)- injected siblings. (v–x) Double-positive HSCs (white arrowheads) inkdrl:RFP; cmyb:EGFPtransgenics in the fgfr4 morphants (x) compared with uninjected (v) and mismatched control MO injected (w) controls. (y) Quantitation of 50 hpfcmyb+kdrl+double-positive HSCs in the DA of fgfr4 morphants (v–x) (uninj,n=5; control MO,n=5; fgfr4 morphants,n=9; *P<0.01, significantly different from uninjected and control MO-injected ones, Student’st-test). Scale bar=100 μm. Figure 7: Fgfr4 is required for somitic dlc expression and HSC specification. ( a – f ) Single-plane confocal images of two-colour FISH for fgfr1 ( a ), dlc ( b ) and merged comparison ( c ), and fgfr4 ( d ), dlc ( e ) and their merged comparison ( f ) at 15 hpf. Yellow arrows indicate expressions of fgfr1 ( a ) or fgfr4 ( d ) in the somites. ( g – u ) Expression of somitic dlc at 15 hpf. ( g – i ), runx1 at 26 hpf ( j – l ), cmyb at 36 hpf ( m – o ), the endothelium marker kdrl ( p – r ) and the aortic marker efnb2a ( s – u ) at 26 hpf in fgfr4-MO2 injected embryos, compared with uninjected and mismatched control MO (fgfr4-CoMO2)- injected siblings. ( v – x ) Double-positive HSCs (white arrowheads) in kdrl:RFP; cmyb:EGFP transgenics in the fgfr4 morphants ( x ) compared with uninjected ( v ) and mismatched control MO injected ( w ) controls. ( y ) Quantitation of 50 hpf cmyb + kdrl + double-positive HSCs in the DA of fgfr4 morphants ( v – x ) (uninj, n =5; control MO, n =5; fgfr4 morphants, n =9; * P <0.01, significantly different from uninjected and control MO-injected ones, Student’s t -test). Scale bar=100 μm. Full size image Although roles for FGF signalling in primitive haematopoiesis have been described [21] , [22] , [23] , its potential function in the embryonic development of HSCs has not been addressed. Here, we demonstrate that FGF signalling is required for HSC specification through its actions in neighbouring somitic tissues. Our studies suggest that FGF signalling in the somite serves to bridge a signalling cascade between a non-canonical Wnt ligand, Wnt16, and the Notch pathway through its regulation of Dlc ( Fig. 8 ). 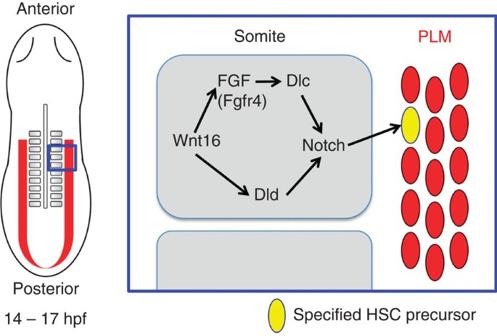Figure 8: Model of the early FGF requirement in HSC specification. Cartoon depicts a dorsal view during mid-somitogenesis (14–17 hpf). FGF signalling specifies HSCs by relaying signals between Wnt16 and Dlc in the somite. Fgfr4 is the key receptor that mediates this Wnt16/Notch HSC specification pathway. Figure 8: Model of the early FGF requirement in HSC specification. Cartoon depicts a dorsal view during mid-somitogenesis (14–17 hpf). FGF signalling specifies HSCs by relaying signals between Wnt16 and Dlc in the somite. Fgfr4 is the key receptor that mediates this Wnt16/Notch HSC specification pathway. Full size image Inhibition of FGF signalling using inducible transgenic hsp70:dn-fgfr1 animals reveals that induction of dn-Fgfr1 at 12 hpf led to significantly fewer specified HSCs. Our strategy for time-specific FGF inhibition allowed us to bypass earlier known requirements for FGF signalling in mesoderm patterning and primitive haematopoiesis [23] , [30] , [44] , [45] , and directly examine the later time points proximal to HSC specification. These results define a critical requirement for FGF signalling in HSC specification from 14 to 17 hpf during somitogenesis, after its role in mesoderm formation and primitive blood cell development has passed. Interestingly, as presented in the companion paper [46] , even later modulation of the FGF pathway at 20.5 hpf shows an opposite role for FGF signalling, limiting emergence of HSCs from the aortic floor. Our studies indicate that FGF signalling during somitogenesis mediates Wnt16 activation of Dlc within the somite, while our collaborators demonstrate that FGFs negatively regulate HSC formation by restricting a necessary pro-haematopoietic BMP signal at 20.5 hpf. Together with past work, these results demonstrate that the regulation of HSC formation by FGF signalling is dynamic, with multiple independent roles present in distinct temporal windows. Sonic Hedgehog (Shh) and Vegf play key roles in patterning the DA and regulating emergence of HSCs. During early zebrafish somitogenesis, Shh activates expression of Vegf that in turn is required for the expression of Notch1 in the arterial vasculature [31] , [47] , [48] . Notch1 is required cell autonomously in the haemogenic endothelium for HSC specification [15] . Our current studies indicate that Fgf signalling does not interact with this pathway. Expression of shh , as well as its targets ptc1 and ptc2 , was not altered following ablation of FGF signalling. No alteration of vegfa was observed in somites of FGF-inhibited embryos, and, conversely, the FGF target pea3 was normal in embryos treated with Vegf inhibitors. Moreover, not only did the vasculature develop morphologically normally, endothelial expression of the Notch ligands dlc and dll4 , as well as the receptors notch1b and notch3 , was normal in the absence of FGF signalling. Our results thus indicate that the requirement for FGF signalling in HSC specification is independent of the Shh and Vegf pathways, but rather operates temporally in parallel. A growing body of evidence supports the idea that gene expression and patterning within the somites play a critical role in HSC specification, but many details remain mysterious. We previously identified an important role for the non-canonical Wnt ligand, Wnt16 in HSC specification. Loss of Wnt16 led to loss of the two key Notch ligands dlc and dld in the somite. These in turn regulate HSC specification, but whether or not each acts directly on the haemogenic endothelium remains to be determined. Multiple lines of evidence supported the idea that the temporal 14–17 hpf requirement observed for FGF signalling in HSC specification is operational within the formed somites. The FGF targets pea3 and erm are expressed in the somites, but not the PLM; so are the key receptors, fgfr1 and fgfr4 . As the FGF signalling requirement we have defined here does not interact with the Shh/Vegf/Notch pathway, we examined the possibility that it interacts with the Wnt16/Dlc/Dld pathway [28] , which is also operational within the somites. Knockdown of Wnt16 reduces the expression of pea3 and fgfr4 , and this loss of expression could be rescued by enforced activation of FGF signalling, revealing Wnt16 is required to turn on or potentiate somitic FGF signalling. These results reveal a novel non-canonical Wnt/Fgf signalling axis upstream of HSC specification. To better locate where FGF signalling acts in the Wnt16/Dlc/Dld/HSC specification pathway, we examined the ability of Fgf to regulate expression of the pivotal somitic Notch ligands dlc and dld . This possibility seemed plausible, given previous studies that have suggested that somitic Notch ligand expression is regulated by FGF signalling [41] . Interestingly dlc , but not dld , requires FGF signalling downstream of Wnt16. We have determined that the key FGFR in this pathway is Fgfr4. Although both fgfr1 and fgfr4 are expressed in the somites, only fgfr4 expression directly overlaps that of dlc , and only knockdown of Fgfr4 has significant effects on dlc expression. Our results strongly suggest the possibility that Fgfr4 cell autonomously regulates expression of Dlc, but we cannot exclude the possibility of paracrine relay signalling within the Fgfr4 + population. Consistent with the notion that Fgfr4 is active within the somites and not in the endothelium, knockdown of Fgfr4 yields changes in somitic but not vascular gene expression, leaving endothelial and arterial markers intact. Importantly, our results locate a requirement for FGF signalling within a now better-defined somitic Wnt16/FGF/Notch HSC specification pathway. FGF signalling here works to activate expression of dlc but not dld , which represents a parallel input downstream of Wnt16, but not evidently regulated through FGF. runx1 + HSCs are partially lost in FGF-inhibited conditions and this loss can be rescued by injection of dlc mRNA. Consistent with the bifurcation of the pathways downstream of Wnt16 at the point of FGF signalling, HSCs are partially ablated in the absence of FGF signalling, and fully ablated when dld is knocked down in parallel to FGF inhibition. The identification of Fgfr4 as a receptor specifically required for HSC generation begs the question of which FGF ligands are active in this process. Our results demonstrate that Wnt16 is critical for cellular reception of the FGF signal, by activating expression of fgfr4 , but do not exclude the possibility that it also activates expression of key ligands and downstream signals transduction factors. The FGF ligands FGF1, FGF8 and FGF17 are expressed in developing somites [49] , [50] , [51] . FGF1 increases the generation of long-term repopulating HSCs in vitro [25] and is required for primitive haematopoiesis in zebrafish embryos [49] . FGF8 has a critical role in mesoderm formation and patterning [52] , [53] and zebrafish studies with fgf8 mutant animals ( ace ) indicate that FGF8 is required for somitogenesis [50] . Likewise, FGF17 potentially plays a role in somite patterning [51] . However, because each of these ligands also has earlier developmental functions, published loss-of-function studies were limited in determining the role of FGFs during the later developmental stages important for haematopoietic specification. Therefore, inducible genetic tools are necessary to further analyse individual roles of FGF ligands in HSC specification. Although our studies have precisely defined a specific temporal window of somitic signalling required for HSC specification, the relay factors that signal to the adjacent PLM to specify HSC precursors remain to be defined. Multiple studies have now defined specific genetic perturbations in which both sclerotome and HSC specification are abrogated, suggesting the possibility that HSC specification somehow requires the sclerotome. The sclerotome is the ventromedial compartment of developing somites, which gives rise predominantly to elements of the axial skeleton. Sclerotome has been postulated to also give rise to the vascular smooth muscle cells (VSMCs) that sheath the dorsal aorta [54] , [55] , [56] , [57] , but others have found a different origin [58] . Similar to wnt16 morphants, and loss of function in either or both of the Notch ligands Dlc and Dld [28] , loss of FGF signalling by either global ablation or specific knockdown of Fgfr4 led to loss of sclerotomal tissues, suggesting that the Wnt16-FGF-Notch signalling cascade in the somite directs sclerotome development that may subsequently relay necessary signals from the somites to the PLM. Our recent results suggest that one such relay signal is another iteration of Notch signalling, where Notch ligands presented by the sclerotome make direct contact with the shared vascular precursors of HSCs as they migrate to form the pre-aortic vascular cord [59] . In addition, subsequent signals may be carried by VSMC precursors derived from the sclerotome [1] . To further address the role of the sclerotome, more tissue-specific transgenic reagents will be necessary to investigate its function and behaviour during HSC development. A second population of somite-derived cells has recently been described that has been suggested to be required for HSC specification, the ‘endotome’, a pax3 + population near the septa (vertical somite boundaries), which incorporates into the maturing endothelium [60] . A similar population has previously been described in chick [61] and possibly mouse [55] , but was not previously implicated in HSC specification. The Wnt16/FGF/Notch pathway appears to be discrete from the endotomal pathway, most notably in that the affected regions of the somite are different ( foxc1b + sclerotome versus pax3 + septa), but we cannot rule out the possibility that Wnt16/FGF/Notch regulates both endotomal and sclerotomal contributions to HSC specification. The fact that in choker mutants, which display an increased contribution of somite-derived cells to the endothelium of the dorsal aorta, wnt16 expression is nearly ablated suggests that the choker mutation ( meox1a ) short circuits the requirement for Wnt16 (ref. 60 ), for example by leading to an upregulation of FGF signalling or enhanced presentation of Notch ligands. In conclusion, our studies suggest that FGF signalling through Fgfr4 is required to mediate a signalling cascade between Wnt16 and Dlc in the developing somite to specify HSCs. These findings provide a better understanding of HSC ontogeny and have elucidated a novel set of regulatory inputs necessary for HSC development. Importantly, our findings shed light on pathways that can be potentially modulated to instruct in vitro production of HSCs from pluripotent precursors, a process that has proven to be extremely challenging. Zebrafish husbandry Wild-type AB* and transgenic hsp70:dn-fgfr1 (Tg(hsp70l:dnfgfr1-EGFP) pd1 ) [27] , ( Tg(cmyb:EGFP) zf169 ) [62] , ( Tg(kdrl:RFP) la4 ) [63] , hsp70:ca-fgfr1 ( Tg(hsp70l:Xla.fgfr1, cryaa:DsRed) pd3 ) [40] , UAS:NICD-myc ( Tg(5xUAE-E1b:6xMYC-notch1a) kca3 ) [42] , hsp70:gal4 ( Tg(-1.5hsp70l:Gal4 )kca4 ) [42] , fli1:EGFP ( Tg(fli1a:EGFP) y1 ) [64] , α-actin:GFP ( Tg(actc1b:GFP) zf13 ) [65] zebrafish embryos and adult fish were raised in a circulating aquarium system (Aquaneering) at 28 °C and maintained in accordance with UCSD Institutional Animal Care and Use Committee (IACUC) guidelines. For heat-shocking transgenic embryos, hsp70:dn-fgfr1 and hsp70:ca-fgfr1 embryos were placed in E3 fish water in a 125-ml flask and transferred to a 38 °C water bath for 20 at 12, 15 or 17 hpf. For double heat-shock of hsp70:gal4 ; UAS:myc-Notch1a-intra ; hsp70:dn-fgfr1 transgenics, embryos in E3 water in a 125-ml flask were incubated in a 38 °C water bath for 20 min at 12 hpf, followed by a 45 min incubation in a 38 °C water bath at 15 hpf. WISH Whole-mount single or double enzymatic in situ hybridization was performed on embryos fixed overnight with 4% paraformaldehyde (PFA) in phosphate buffered saline (PBS). Fixed embryos were washed briefly in PBS and transferred stepwise into methanol in PBS for storage at −20 °C. Embryos were rehydrated stepwise through methanol in PBS–0.1% Tween 20 (PBT). Rehydrated embryo samples were then incubated with 10 μg ml −1 proteinase K in PBT for 5 min for 5 to 10 somite stage (12–15 hpf) embryos and 15 min for 24 to 36 hpf embryos. After proteinase K treatment, samples were washed in PBT and refixed in 4% PFA for 20 min at room temperature. After washes in two changes of PBT, embryos were prehybridized at 65 °C for 1 h in hybridization buffer (50% formamide, 5x SSC, 500 μg ml −1 torula (yeast) tRNA, 50 μg ml −1 heparin, 0.1% Tween 20, 9 mM citric acid (pH 6.5)). Samples were then hybridized overnight in hybridization buffer including digoxigenin (DIG)- or fluorescein-labelled RNA probe. After hybridization, experimental samples were washed stepwise at 65 °C for 15 min each in hybridization buffer in 2 × SSC mix (75%, 50%, 25%), followed by two washes with 0.2 × SSC for 30 min each at 65 °C. Further washes were performed at room temperature for 5 min each with 0.2 × SSC in PBT (75%, 50%, 25%). Samples were incubated in PBT with 2% heat-inactivated goat serum and 2 mg ml −1 bovine serum albumin (block solution) for 1 h and then incubated overnight at 4 °C in block solution with diluted DIG-antibodies (1:5,000) conjugated with alkaline phosphatase (AP) (Roche). To visualize WISH signal, samples were washed three times in AP reaction buffer (100 mM Tris, pH 9.5, 50 mM MgCl 2 , 100 mM NaCl, 0.1% Tween 20, 1 mM levamisole (Sigma)) for 5 min each and then incubated in the AP reaction buffer with NBT/BCIP substrate (Promega). For double enzymatic WISH, the processed samples were washed in 0.1 M glycine (pH 2.2) for 20 min and then washed in PBT for 5 min. After storing washed samples in methanol for 1 h, the embryos samples were stepwise rehydrated in methanol in PBT for 5 min each (75%, 50%, 25%) and further washed in PBT. After incubation in block solution for 1 h, the samples were incubated overnight at 4 °C in block solution with diluted fluorescein antibodies (1:5,000) conjugated with AP (Roche). After PBT washes, the samples were washed two times in 0.1 M Tris-HCl (pH 8.2). Embryos were then incubated in 0.1 M Tris-HCl (pH 8.2) with Fast Red Tablets (Roche). After obtaining red signals, embryos were washed in 0.1 M Tris-HCl (pH 8.2) and refixed in 4% PFA. For two-colour double FISH, embryos were blocked in maleic acid buffer (MAB; 150 mM maleic acid, 100 mM NaCl, pH 7.5) with 2% Roche blocking reagent (MABB) for 1 h at room temperature, after hybridizing at 65 °C with probes as described above. Embryos were incubated overnight at 4 °C in MABB with anti-fluorescein POD (Roche) at a 1:500 dilution. After four washes in MAB for 20 min each followed by washes in PBS at room temperature, embryo samples were incubated in TSA Plus Fluorescein Solution (Perkin Elmer) for 1 h. Embryos were washed 10 min each in methanol in PBS (25%, 50%, 75%, 100%). Embryos were incubated in 1% H 2 O 2 in methanol for 30 min at room temperature and washed for 10 min each in methanol in PBS (75%, 50% 25%) and 10 min in PBS. After blocking for 1 h in MABB, embryos were incubated overnight at 4 °C in MABB with anti-DIG POD (Roche) at a 1:1,000 dilution. Samples were washed and incubated in TSA Plus CY3 solution (Perkin Elmer) as described above. Embryos were washed three times for 10 min each in PBT and refixed in 4% PFA after the staining was complete. Antisense RNA probes for the following genes were prepared using probes containing DIG or fluorescein labelled UTP: runx1 , cmyb , rag1 , pea3 , er m , scl , lmo2 , cdx4 , shh , desma , kdrl , cdh5 , gata1 , l-plastin , efnb2a , fli1 , fgfr1 , fgfr2 , fgfr3 , fgfr4 , dlc , dld , dll4 , notch1b , notch3 , wnt16 , foxc1b. Immunofluorescence and microscopy For immunofluorescence staining for Myc in hsp70:gal4 ; UAS:NICD-myc zebrafish embryos after WISH, 100% acetone was added to the embryos (7 min at −20 °C) instead of proteinase K during the WISH procedure described above. WISH samples of embryos were blocked in MABB for 1 h and incubated overnight in MABB with anti-Myc monoclonal 9E10 antibodies at 1:100 (Covance). After four washes in MABB for 30 min each, embryos were incubated in Dylight 488 AffiniPure donkey anti-mouse IgG secondary antibodies (Jackson Immunoresearch Laboratories) at 1:100 in MABB. After staining, embryos were washed in MABB for four times for 30 min each. The samples were imaged using a stereo zoom microscope (Zeiss, Axio Zoom). Live hsp70:dn-fgfr1 and kdrl:RFP; cmyb:EGFP transgenic embryos and flat-mount or whole-mount two-colour double FISH samples were imaged using confocal microscopy (Leica, SP5). GFP and fluorescein were excited by a 488-nm laser, while DsRed and CY3 were excited by 543 nm. Pharmacological treatment SU5402 (Calbiochem) and ZM306416 (Tocris) was dissolved in DMSO at a concentration of 10 mM. Zebrafish AB* embryos were incubated in 5 ml of 5 μM SU5402 solution from 12 to 15 hpf and 5 μM ZM306416 solution from 10 hpf in the dark, followed by fixation with 4% PFA. Microinjections of morpholinos and mRNA Antisense morpholinos (MOs; Gene Tools, LLC) were diluted as 1 or 3 mM stock in DEPC-treated H 2 O. 5 ng of standard control MO (St.CoMO) [66] , wnt16-MO [28] , dld-MO2 (ref. 28 ), fgfr1-MO1 (ref. 67 ), fgfr4-MO1 [68] , fgfr4-CoMO2 and fgfr4-MO2 were injected at the 1- to 2-cell stage of development. The sequence of translation-blocking targeted fgfr4-MO2 is 5′- AGATGCTCAACATCTTGCTGAGGTA -3′ and 5 base pair mismatched fgfr4 control MO2 (fgfr4-CoMO2) is 5′- AaATGaTCAAaATCTTaCTGAaGTA -3′ (lower case letter indicates mismatched base pairs). Full-length dlc mRNA was synthesized from linearized pCS2+ dlc [28] with the mMessege mMaching kit (Ambion). dlc mRNA was injected with 100 pg into 1- to 2-cell stage hsp70 : dn - fgfr1 transgenic embryos for rescue experiments. All microinjections were performed with the indicated concentration of RNA or MO in a volume of 1 nl using a PM 1,000 cell microinjector (MDI). FACS fli1:EGFP and α-actin:GFP embryos (~50 embryos each) at 17 hpf were dissociated in PBS by homogenizing with sterile plastic pestle or pipette. Dissociated cells were filtered through a 40-μm nylon cell strainer (Falcon 2340) and then rinsed with PBS with 1% fetal bovine serum. Propidium iodide (Sigma) was added (1 μg ml −1 ) to exclude dead cells and debris. FACS was performed based on GFP fluorescence [5] with a FACS Aria II flow cytometer (Beckton Dickinson). Quantitative real-time PCR Total RNA was collected from posterior trunk of the embryos or whole embryos (~30 embryos) using TRIzol reagent (Ambion, Life Technologies) and isolated fli1:EGFP + and α-actin:GFP + cells with the RNeasy kit (Qiagen). cDNA was generated from total RNA with iScript cDNA synthesis kit (Bio Rad). The following primers were used for cDNA quantification: ef1α (forward, 5′- GAGAAGTTCGAGAAGGAAGC -3′; reverse, 5′- CGTAGTATTTGCTGGTCTCG -3′) [33] , runx1 (forward, 5′- CGGTGAACGGTTAATATGAC -3′; reverse, 5′- CTTTTCATCACGGTTTATGC -3′) [33] , kdrl ( forward , 5 ′- CTCCTGTACAGCAAGGAATG -3′; reverse, 5′- ATCTTTGGGCACCTTATAGC -3′) [5] , erm ( forward, 5′- GGTGCCTCCAAATAAGTCTC -3′, reverse 5′- TGGAAATCTGGAACAAACTG -3′), efnb2a (forward, 5′- CCCATTTCCCCCAAAGACTA -3′; reverse, 5′- CTTCCCCATGAGGAGATGC -3′), fgfr1 (forward, 5′- AGTGATGTGGAGTTCGAGTG -3′; reverse, 5′- CAAGCAGGTGTACTCTCCAG -3′) and fgfr4 (forward, 5′- CAAACAACTTGTGGAAGAGC -3′; reverse, 5′- AGCATCATGGGTAAACACAG -3′). How to cite this article: Lee, Y. et al . FGF signalling specifies haematopoietic stem cells through its regulation of somitic Notch signalling. Nat. Commun. 5:5583 doi: 10.1038/ncomms6583 (2014).